An ALS-associated mutation in the FUS 3′-UTR disrupts a microRNA–FUS regulatory circuitry While the physiologic functions of the RNA-binding protein FUS still await thorough characterization, the pathonegetic role of FUS mutations in amyotrophic lateral sclerosis (ALS) is clearly established. Here we find that a human FUS mutation that leads to increased protein expression, and was identified in two ALS patients with severe outcome, maps to the seed sequence recognized by miR-141 and miR-200a in the 3′-UTR of FUS. We demonstrate that FUS and these microRNAs are linked by a feed-forward regulatory loop where FUS upregulates miR-141/200a, which in turn impact FUS protein synthesis. We also show that Zeb1, a target of miR-141/200a and transcriptional repressor of these two microRNAs, is part of the circuitry and reinforces it. Our results reveal a possible correlation between deregulation of this regulatory circuit and ALS pathogenesis, and open interesting perspectives in the treatment of these mutations through ad hoc- modified microRNAs. Amyotrophic lateral sclerosis (ALS) is a late-onset neurodegenerative disease that leads to specific degeneration of upper and lower motoneurons and to progressive paralysis. Most patients with ALS die by respiratory failure within 3–5 years after symptoms onset [1] . When patients have affected relatives, they are classified as familial ALS cases, otherwise they are considered as sporadic ALS ones. Familial ALS accounts for 5–10% of all patients and several genes have been identified that, in their mutant forms, account for the onset of the disease [2] . On the other side the causes of sporadic ALS are still unknown. Mutations in FUS (Fused in Sarcoma, also known as, Translocated in Liposarcoma (TLS)), an RNA-binding protein involved in several different processes of RNA biogenesis and maturation [3] , have been found in 4% of familial cases of ALS [4] , [5] . Pathogenic mutations in FUS were identified in several domains of the protein, with the majority found in the glycine-rich region and within the nuclear localization signal, the latter being required for proper nuclear localization [6] . Most of these mutations alter the subcellular partitioning of the protein, which leads to a decrease of the nuclear content and an increase in the cytoplasm. Notably, recent sequencing of the 3′-untranslated region (3′-UTR) of FUS messenger RNA (mRNA) in 420 ALS patients, negative for mutations in the currently known ALS-associated genes, identified four mutations linked to severe outcomes that caused a strong increase in FUS accumulation [7] . The pathogenetic effects of wild-type (wt) FUS overexpression observed in these patients suggests that not only the nuclear–cytoplasmic imbalance of the mutant protein, but also alteration of the physiological levels of the wt protein may contribute to ALS pathogenesis. In agreement with this, transgenic mice overexpressing wt human FUS were shown to develop ALS with an aggressive phenotype [8] . The findings that both reduced and increased levels of FUS are associated with the ALS phenotype point to the importance of a tight control of FUS expression to ensure correct cellular homeostasis [8] , [9] , [10] . Along this line, the identification of mutations affecting the regulation of FUS expression opens interesting new perspectives in the study of FUS regulation in ALS pathogenesis. In this study, we describe that one of the 3′-UTR mutations (G48A) affects the binding site of miR-141/200a, thus making FUS mRNA insensitive to the repression of these microRNAs (miRNAs). We also show that FUS is an activator of miR-141/200a biogenesis, indicating the existence of a feed-forward regulatory loop between these components. Zinc-finger E-box-binding homeobox 1 (Zeb1), a target of miR-141/200a and transcriptional repressor of these two miRNAs, has been identified as an additional member of the circuitry and shown to reinforce it. Our results suggest a possible link between the alteration of this regulatory loop, determined by the G48A mutation, and ALS pathogenesis. The role of 3′-UTR in FUS regulation In order to analyse the contribution of non-coding regions in FUS regulation, a RFP–FUS fusion complementary DNA (cDNA) copy, devoid of the 3′-UTR, was overexpressed in SK-N-BE neuroblastoma cells. The absence of the 3′-UTR resulted in a strong accumulation of the RFP–FUS fusion protein alongside a conspicuous reduction in endogenous FUS mRNA ( Supplementary Fig. 1a ) and protein ( Fig. 1a ). This observation suggested the existence of a feedback regulation exerted by the exogenous construct (devoid of introns and 3′-UTR) on expression of endogenous FUS . In agreement with recent observations by Zhou et al. [11] , we also observed that an excess of FUS strongly induced the skipping of exon 7 from the endogenous FUS pre-mRNA ( Supplementary Fig. 1b ). Along this line, the downregulation of FUS through RNA interference resulted in a strong decrease of the exon 7-skipped isoform ( Supplementary Fig. 1c ). FUS exon 7 skipping produces an out-of-frame mRNA unable to make a functional protein [11] . Since exon 7 contains multiple binding sites for FUS itself, it was suggested that FUS might function in the nucleus to control the level of splicing. In this scenario, FUS regulates its own synthesis by preventing exon 7 inclusion [11] . The strong accumulation of the RFP–FUS fusion protein in the absence of its endogenous 3′-UTR ( Fig. 1a ) also suggested a possible role for the 3′-UTR in FUS regulation. 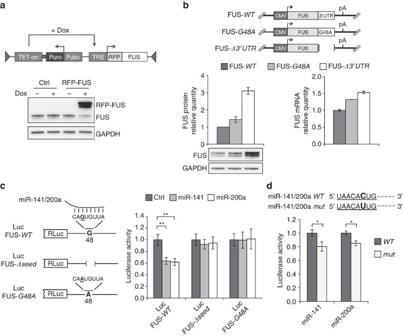Figure 1: Role of the 3′-UTR region in FUS regulation. (a) Upper panel: construct for Dox-inducible expression of a RFP–FUS fusion protein, stably integrated in SK-N-BE cells16. Lower panel: western blot analysis with FUS antibodies on total proteins extracted from SK-N-BE cells, carrying a RFP control construct (Ctrl) or the RFP–FUS expression cassette, grown for 48 h in absence (−) or presence (+) of doxycycline (Dox). GAPDH was used as a loading control. See full blots with marker position inSupplementary Fig. 2a. (b) FUS cDNA constructs utilized; FUS–WT, contains the wild-type 3′-UTR, while the mutant derivatives contain either the G48A substitution (FUS–G48A) or the deletion of the entire 3′-UTR (FUS-Δ3′-UTR). Histograms show the levels of total FUS protein (left panel) and mRNA (right panel) obtained from SK-N-BE cells transfected with the different FUS constructs. FUS mRNA levels were normalized on the neomycin marker co-expressed from the same plasmid. A representative western blot analysis is shown below the corresponding graph. See full blots with marker position inSupplementary Fig. 2b. (c) Left panel: luciferase fusion constructs. The MRE sequence for mir-141/200a is indicated together with the G48A mutation. Right panel: relative luciferase levels of Luc–FUS–WT,Luc–FUS-Δseedand Luc–FUS–G48Aconstructs co-transfected in SK-N-BE cells with an empty vector (Ctrl) or with miRNA (miR-141 or miR-200a)-expressing plasmids. (d) Schematic representation of the seed sequence of miR-141 and miR-200a (miR-141/200aWT) and of their mutant derivatives (miR-141/200amut) containing the complementary substitution to the G48A mutation. Histograms indicate the relative luciferase activity of the Luc–FUS–G48Aconstruct co-transfected in SK-N-BE cells with wild-type (black bars) or mutant (white bars) miRNA-expressing plasmids. Luciferase activity was measured as the ratio between Firefly and Renilla Luciferase activities and shown with respect to a control sample set to a value of 1. In the figure, data were derived from three independent experiments; error bars represent s.e., *P<0.05 corresponds to the one-tailed Student’st-test, **P<0.01. Figure 1: Role of the 3′-UTR region in FUS regulation. ( a ) Upper panel: construct for Dox-inducible expression of a RFP–FUS fusion protein, stably integrated in SK-N-BE cells [16] . Lower panel: western blot analysis with FUS antibodies on total proteins extracted from SK-N-BE cells, carrying a RFP control construct (Ctrl) or the RFP–FUS expression cassette, grown for 48 h in absence (−) or presence (+) of doxycycline (Dox). GAPDH was used as a loading control. See full blots with marker position in Supplementary Fig. 2a . ( b ) FUS cDNA constructs utilized; FUS– WT , contains the wild-type 3′-UTR, while the mutant derivatives contain either the G48A substitution (FUS– G48A ) or the deletion of the entire 3′-UTR (FUS -Δ 3′- UTR ). Histograms show the levels of total FUS protein (left panel) and mRNA (right panel) obtained from SK-N-BE cells transfected with the different FUS constructs. FUS mRNA levels were normalized on the neomycin marker co-expressed from the same plasmid. A representative western blot analysis is shown below the corresponding graph. See full blots with marker position in Supplementary Fig. 2b . ( c ) Left panel: luciferase fusion constructs. The MRE sequence for mir-141/200a is indicated together with the G48A mutation. Right panel: relative luciferase levels of Luc–FUS– WT, Luc–FUS- Δseed and Luc–FUS –G48A constructs co-transfected in SK-N-BE cells with an empty vector (Ctrl) or with miRNA (miR-141 or miR-200a)-expressing plasmids. ( d ) Schematic representation of the seed sequence of miR-141 and miR-200a (miR-141/200a WT ) and of their mutant derivatives (miR-141/200a mut ) containing the complementary substitution to the G48A mutation. Histograms indicate the relative luciferase activity of the Luc–FUS– G48A construct co-transfected in SK-N-BE cells with wild-type (black bars) or mutant (white bars) miRNA-expressing plasmids. Luciferase activity was measured as the ratio between Firefly and Renilla Luciferase activities and shown with respect to a control sample set to a value of 1. In the figure, data were derived from three independent experiments; error bars represent s.e., * P <0.05 corresponds to the one-tailed Student’s t -test, ** P <0.01. Full size image Using a 3′-rapid amplification of cDNA ends (RACE) assay, we established the presence of a single 164-nucleotide-long 3′-UTR in SK-N-BE ( Supplementary Fig. 1d ). To test the contribution of the 3′-UTR on protein accumulation, two different cDNA constructs—with or without this region (FUS– WT and FUS- Δ3′-UTR )—were transfected in SK-N-BE cells and the amount of protein was compared. Figure 1b shows that, in comparison with FUS–WT , the FUS - Δ3′-UTR construct resulted in an increased accumulation of both FUS protein and mRNA. The G48A mutation in FUS 3′-UTR alters miR-141/200a binding Bioinformatics search [12] , [13] for miRNA-responsive elements in the FUS 3′-UTR indicated that among the identified 3′-UTR mutations [7] , two patients carried the G48A substitution (in one case of inherited type), which localizes to a predicted binding site for miR-141 and miR-200a. These two miRNAs share the same seed sequence and belong to the same miRNA family [14] . The miR-200 family includes five members (miR-200a, miR-200b, miR-200c, miR-429 and miR-141) that are encoded at two independent loci: the miR-200b/200a/429 cluster located on chromosome 1, and the miR-200c/141 cluster on chromosome 12. The members of this family are of particular interest for human health and disease, because they have been shown to be downregulated during tumour progression and to act as key regulators of epithelial-to-mesenchymal transition [15] . When the G48A mutation was tested in the context of a cDNA construct ( FUS – G48A ), the levels of FUS protein and mRNA were reproducibly higher with respect to those of the wt construct ( Fig. 1b ), indicating the relevant contribution of this mutation on the control of FUS accumulation. Nevertheless, the increase in FUS protein did not reach the levels observed with the entire deletion of the 3′-UTR (FUS- Δ3′-UTR ), suggesting the presence of additional regulatory elements besides the MRE (miRNA recognition element) for miR-141/200a. This seems indeed to be the case since three other mutations, associated with severe ALS phenotypes and linked to high accumulation of protein, were also identified in this region [7] . However, according to TargetScan and PicTar analyses [12] , [13] , none of those mutations appear to affect conserved miRNA-binding sites. Luciferase reporters harbouring the 3′-UTR of FUS ( Luc–FUS – WT ; Fig. 1c ) or the deletion of the miR-141/200a seed site ( Luc–FUS - Δseed ) or the G48A point mutation ( Luc–FUS – G48A ) were individually co-transfected in SK-N-BE cells with miR-141- and miR-200a-expressing plasmids or with a control plasmid (Ctrl). Luciferase levels in Luc–FUS – WT transfected cells were significantly reduced with each one of the two miRNAs, whereas Luc–FUS - Δseed transfected did not exhibit this effect ( Fig. 1c ). Notably, the Luc–FUS–G48A construct, containing the G48A point mutation, was also insensitive to miR-141 or miR-200a repression ( Fig. 1c ). However, co-transfection of Luc–FUS–G48A with miR-141 or miR-200a derivatives, containing a nucleotide substitution complementary to the G48A mutation (miR-141/200a mut ), resulted in rescue of miRNA-dependent repression ( Fig. 1d ). These data indicate the specificity of the G to A substitution for miR-141/200a recognition and function. miR-141/200a are upregulated on FUS overexpression We next examined the levels of these miRNAs in control and RFP–FUS expressing cells. Interestingly, on FUS overexpression in SK-N-BE cells ( Fig. 1a ) the levels of miR-141 and miR-200a increased ( Fig. 2a ), along with an increase in the levels of the corresponding pri-miRNAs ( Fig. 2b ). In contrast, no upregulation was observed for the miR-15a and miR-432 miRNAs, previously shown to be unaffected by alteration in FUS levels [16] . Moreover, as a consequence of the miR-141/200a increase obtained after Dox induction of flag–FUS , we observed that the Zeb1 —previously reported to be post-transcriptionally repressed by the members of miR-200 family [17] —was downregulated ( Fig. 2c ). Zeb1 has been described as a transcriptional repressor of the two clusters harbouring the miR-200 family by direct binding to common regulatory elements in their promoters [18] , [19] . This, together with the findings reported here, suggested the existence of a circuitry in which an increase in miR-141 and miR-200a upregulates their own expression through the downregulation of Zeb1. miR-141 and miR-200a were also upregulated on FUS – G48A overexpression relative to FUS – WT ( Fig. 2d,e ). It is important to note that in this case, owing to the lower level of FUS upregulation, only a mild effect on these miRNAs was observed. Notably, miR-141 and miR-200a were downregulated by short interfering RNA (siRNA)-mediated FUS knockdown ( Supplementary Fig. 1e ). Altogether, these data indicate a direct correlation between the levels of FUS and those of miR-141/200a. 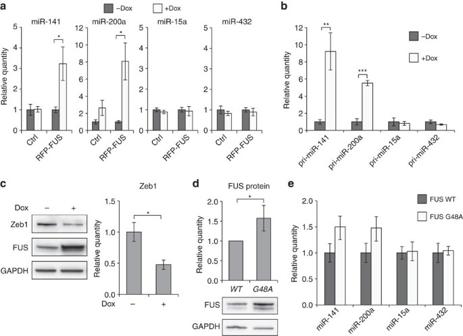Figure 2: Effects of FUS overexpression on miRNA levels. (a,b) Levels of mature and pri-miRNA species for miR-141 and miR-200a measured by quantitative reverse transcriptase (qRT)-PCR in SK-N-BE cells (in absence or presence of Dox) stably transfected with either a RFP control (Ctrl) or RFP–FUS cDNAs. miR-15a and miR-432 as well as their corresponding pri-miRNA molecules were used as controls. Mature miRNA levels were normalized against snoRNA-U25 while pri-miRNAs against pre-GAPDH. (c) Left panel: representative western blot analysis of Zeb1 and FUS expression in SK-N-BE cells expressing Dox-inducible flag-FUS cDNAa. GAPDH was used as loading control. Right panel: densitometric analysis of Zeb1 normalized against GAPDH. See full blots with marker position inSupplementary Fig. 2c. (d) Lower panel: representative western blot analysis of FUS–WTand FUS–G48Aexpression in SK-N-BE cells transfected with the corresponding plasmids. Upper panel: densitometric analysis of FUS–WTand FUS–G48Anormalized against GAPDH. See full blots with marker position inSupplementary Fig. 3a. (e) Levels of miR-141 and miR-200a measured by qRT-PCR in SK-N-BE cells treated as in paneld. miR-15a and miR-432 were used as controls. miRNAs levels were normalized against snoRNA-U44. All data were derived from three independent experiments; error bars represent s.e.m. *P<0.05 corresponds to the one-tailed Student’st-test, **P<0.01, ***P<0.001. Figure 2: Effects of FUS overexpression on miRNA levels. ( a , b ) Levels of mature and pri-miRNA species for miR-141 and miR-200a measured by quantitative reverse transcriptase (qRT)-PCR in SK-N-BE cells (in absence or presence of Dox) stably transfected with either a RFP control (Ctrl) or RFP–FUS cDNAs. miR-15a and miR-432 as well as their corresponding pri-miRNA molecules were used as controls. Mature miRNA levels were normalized against snoRNA-U25 while pri-miRNAs against pre-GAPDH. ( c ) Left panel: representative western blot analysis of Zeb1 and FUS expression in SK-N-BE cells expressing Dox-inducible flag-FUS cDNA a . GAPDH was used as loading control. Right panel: densitometric analysis of Zeb1 normalized against GAPDH. See full blots with marker position in Supplementary Fig. 2c . ( d ) Lower panel: representative western blot analysis of FUS– WT and FUS– G48A expression in SK-N-BE cells transfected with the corresponding plasmids. Upper panel: densitometric analysis of FUS– WT and FUS– G48A normalized against GAPDH. See full blots with marker position in Supplementary Fig. 3a . ( e ) Levels of miR-141 and miR-200a measured by qRT-PCR in SK-N-BE cells treated as in panel d . miR-15a and miR-432 were used as controls. miRNAs levels were normalized against snoRNA-U44. All data were derived from three independent experiments; error bars represent s.e.m. * P <0.05 corresponds to the one-tailed Student’s t -test, ** P <0.01, *** P <0.001. Full size image FUS controls miR-141/200a biogenesis FUS was previously described as a Drosha interactor [20] and shown to enhance miRNA expression by direct binding to nascent pri-miRNAs on chromatin and facilitating co-transcriptional processing [16] , [21] . To dissect the mechanism by which FUS affects miR-141/200a biogenesis, we therefore tested these features on miR-141 and miR-200a. 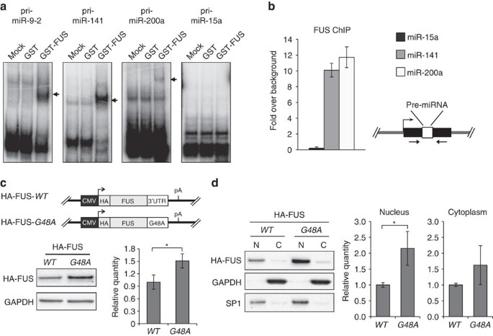Figure 3: FUS binds pri-miRNAs and controls their biogenesis. (a) Gel mobility-shift assay using the indicatedin vitro32P-labelled pri-miRNA transcripts with either GST or GST–FUS recombinant proteins16. The arrows point to the specific RNA–protein complexes. (b) Chromatin immunorecipitation (ChIP) analysis with FUS antibodies on chromatin from SK-N-BE cells expressing Dox-inducible flag–FUS cDNA16. Genomic regions coding for miR-141, miR-200a and miR-15a were analysed using primers that amplify the pri-miRNA-containing regions, as schematically shown. Co-amplifications were carried out with primers specific for miRNA and the chromosome 4 intergenic region. The histograms show the immunorecipitation values on miRNA loci normalized for the intergenic region and expressed as enrichment over background signals (immunoglobulin G). (c) Upper panel: schematic representation of the constructs HA–FUS–WTand HA–FUS–G48A. Lower panels: representative western blot analysis on total protein extract from SK-N-BE transfected with the above constructs. Anti-HA antibodies were used for both HA–FUS–WTand HA–FUS–G48Adetection while GAPDH was used as a loading control. On the right the densitometric analysis for HA–FUS–WTand HA–FUS–G48Anormalized against GAPDH is shown. See full blots with marker position inSupplementary Fig. 3b. (d) Left panel: representative western blot analysis on nuclear (N) and cytoplasmic (C) fractions from SK-N-BE treated as in panelc. Anti-HA antibodies were used for both HA–FUS–WTand HA–FUS–G48Adetection while GAPDH and SP1 were used as loading controls for cytoplasmic and nuclear compartments. Right panel: the histograms show the densitometric analysis for both HA–FUS–WTand HA–FUS–G48Aproteins in the nucelar and cytoplasmic fractions normalized against SP1 and GAPDH, respectively. See full blots with marker position inSupplementary Fig. 4a. All data were derived from three independent experiments; error bars represent s.e.m., *P<0.05 corresponds to the one-tailed Student’st-test. Figure 3a shows that FUS interacts in vitro with both pri-miR-141 and pri-miR-200a. Specific binding also occurs with the positive control pri-miR-9-2, while no interaction is observed with the negative control, pri-miR-15a [16] . According to previous data indicating the chromatin localization of FUS [16] , chromatin immunorecipitation with anti-FUS antibodies revealed a specific localization of FUS on the chromosomal loci encoding for miR-141 and miR-200a, while no localization was detected on the negative control, miR-15a ( Fig. 3b ). Figure 3: FUS binds pri-miRNAs and controls their biogenesis. ( a ) Gel mobility-shift assay using the indicated in vitro 32 P-labelled pri-miRNA transcripts with either GST or GST–FUS recombinant proteins [16] . The arrows point to the specific RNA–protein complexes. ( b ) Chromatin immunorecipitation (ChIP) analysis with FUS antibodies on chromatin from SK-N-BE cells expressing Dox-inducible flag–FUS cDNA [16] . Genomic regions coding for miR-141, miR-200a and miR-15a were analysed using primers that amplify the pri-miRNA-containing regions, as schematically shown. Co-amplifications were carried out with primers specific for miRNA and the chromosome 4 intergenic region. The histograms show the immunorecipitation values on miRNA loci normalized for the intergenic region and expressed as enrichment over background signals (immunoglobulin G). ( c ) Upper panel: schematic representation of the constructs HA–FUS– WT and HA–FUS– G48A . Lower panels: representative western blot analysis on total protein extract from SK-N-BE transfected with the above constructs. Anti-HA antibodies were used for both HA–FUS –WT and HA–FUS– G48A detection while GAPDH was used as a loading control. On the right the densitometric analysis for HA–FUS –WT and HA–FUS– G48A normalized against GAPDH is shown. See full blots with marker position in Supplementary Fig. 3b . ( d ) Left panel: representative western blot analysis on nuclear (N) and cytoplasmic (C) fractions from SK-N-BE treated as in panel c . Anti-HA antibodies were used for both HA–FUS –WT and HA–FUS– G48A detection while GAPDH and SP1 were used as loading controls for cytoplasmic and nuclear compartments. Right panel: the histograms show the densitometric analysis for both HA–FUS –WT and HA–FUS– G48A proteins in the nucelar and cytoplasmic fractions normalized against SP1 and GAPDH, respectively. See full blots with marker position in Supplementary Fig. 4a . All data were derived from three independent experiments; error bars represent s.e.m., * P <0.05 corresponds to the one-tailed Student’s t -test. Full size image One obvious assumption to explain FUS activity was that it could facilitate co-transcriptional microprocessor activity. To test this possibility, in vitro -processing extracts were produced from SK-N-BE cells and supplemented with recombinant FUS protein. The addition of recombinant FUS produces a very slight but reproducible increase of pri-miR-141 conversion into the pre-miRNA form ( Supplementary Fig. 1f ). The mild effect observed likely reflects the fact that the in vitro system does not allow the proper reconstitution of the process owing to template structural problems or the absence of additional factors acting in vivo . Also, owing to the described role of FUS in transcription [22] and in consideration of the observed upregulation of the pri-miRNA species, we cannot rule out the possibility of a more complex effect at the level of transcription. Moreover, as indicated above, part of the increase in miR-141/200a biogenesis could be a result of the downregulation of Zeb1. Finally, to demonstrate that the G48A mutation indeed results in increased FUS protein in the nuclear compartment, and to be able to distinguish the exogenous from the endogenous protein, we used HA–FUS constructs carrying either the wt 3′-UTR ( HA–FUS – WT ) or the G48A mutant derivative ( HA–FUS – G48A ). The results indicate that the rise in FUS protein ( Fig. 3c ), derived from the 3′-UTR mutant construct produces a specific increase in nuclear FUS protein ( Fig. 3d ). The increase in FUS protein therefore occurs in the proper cellular compartment to affect miRNA synthesis. In this study, we provide evidence for the existence of a feed-forward regulatory loop in which FUS increases the expression levels of two miRNAs, which in turn regulate FUS accumulation. Moreover, we extended this circuitry with the identification of Zeb1, another target of miR-141/200a, which is a transcriptional repressor of both miRNAs. Zeb1 indeed undergoes downregulation when the levels of FUS increase ( Fig. 4 ). Altogether, these data indicate that homeostatic levels of FUS depend on a tight control exerted by a complex network of factors functionally interconnected among each other ( Fig. 4 ). Interestingly, we show that one mutation found in two ALS patients affects this pathway, thus suggesting a potential link with ALS pathogenesis and pointing to the possibility that these type of mutations produce pleiotropic consequences. 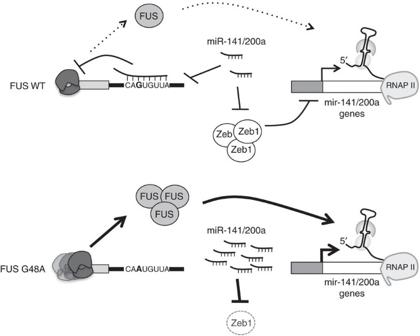Figure 4: Proposed model for FUS and miR-141/200a regulatory circuitry. Schematic representation of the positive feed-forward control loop linking FUS, miR-141/200a and Zeb1 (upper panel). Mutations in the miR-141/200a recognition element in the 3′-UTR of FUS determines the exit from the circuitry with increase of FUS and the miRNAs in parallel to decrease of Zeb1 (lower panel). Figure 4: Proposed model for FUS and miR-141/200a regulatory circuitry. Schematic representation of the positive feed-forward control loop linking FUS, miR-141/200a and Zeb1 (upper panel). Mutations in the miR-141/200a recognition element in the 3′-UTR of FUS determines the exit from the circuitry with increase of FUS and the miRNAs in parallel to decrease of Zeb1 (lower panel). Full size image The increase of miR-200a as a consequence of the disruption of the regulatory loop is quite interesting since its upregulation was described to occur in different neurodegenerative diseases, such as Alzheimer [23] and Huntington [24] . Moreover, miR-200a-predicted targets were implicated in regulating synaptic function, neurodevelopment and neuronal survival [24] , suggesting that deregulation of miR-200a, as a consequence of FUS mutation, might have an impact on ALS pathogenesis. It is clear from our data that to induce alteration of the circuitry indicated in the model, imbalance of one of the components should be achieved. With high levels of FUS protein (obtained with a construct devoid of the entire 3′-UTR), the circuitry is easily altered with a strong increase in miR-141/200a and Zeb1 downregulation. In the case of the G48A mutation, only a small increase in FUS protein is obtained and, as a consequence, the effect on miR-141/200a levels is limited. However, we propose that this is important for explaining the ALS pathology in which, despite the ubiquitous expression of FUS , only motoneurons are affected. Considering the slight effect of the G48A mutation, we believe that the alteration of the circuitry becomes pathogenetically relevant only at long times and in post-mitotic cells such as motoneurons, where accumulation effects are relevant, while otherwise not affecting proliferating cells. However, confirmation of the direct link between the FUS/miR-141/200a circuitry and ALS pathogenesis can only be obtained from analysis of the expression levels of the different components in the context of the heterozygotic G48A genetic background. Finally, we show that the G48A mutation can be suppressed by modified miRNAs, suggesting the possibility of restoring proper FUS level, opening new avenues for the treatment of this type of mutations. Oligonucleotides Oligonucleotide sequences used in this study are listed in Supplementary Table 1 . Cell cultures and treatments SK-N-BE(2)-C cells, from ATCC (Cat. No. CRL-2268), were cultured in RPMI medium 1640 (Gibco) supplemented with 10% fetal bovine serum, L -glutamine and penicillin/streptomycin (Gibco). The cell lines were transfected using Lipofectamine and Plus Reagent (Invitrogen) and induced to differentiate with 10 μM all-trans-retinoic acid (Sigma-Aldrich) [25] . SiRNAs targeting the FUS-coding region (Hs_FUS_4 FlexiTube siRNA, SI00070518, Qiagen) were transfected using HiPerfect Transfection Reagent (Qiagen) according to the manufacturer’s instructions. For the generation of stable SK-N-BE cells expressing FUS protein, upon plasmid transfection (epB-Puro-TT-derived plasmids and epiggyBac transposase vector) the cells were selected by Puromycin (1 μg ml −1 ) treatment and the expression of the different forms of FUS protein was induced by adding Doxycycline (0,2 μg ml −1 ) to the culture medium for 48 h. Plasmid construction To generate the constructs overexpressing miRNAs, the genomic fragments containing pri-miR-141 and pri-miR-200a were PCR amplified from human and mouse genomic DNA, respectively, (all oligonucleotides used in this study are listed in Supplementary Table 1 ) and cloned using Bgl II and Xho I restriction sites of U1snRNA expression cassette [26] . The mutant plasmids overexpressing miR-141 mut and miR-200a mut were obtained by double inverse PCR amplification on the previous cloned plasmids to obtain the single-point mutation of the mature miRNAs, and the complementary substitution for rescuing a correct conformation of the pri-miRNA structure for the efficient processing (oligonucleotides are listed in Supplementary Table 1 ). epB-Puro-TT-derived plasmids for overexpressing RFP, RFP–FUS and flag–FUS fusion cDNAs are described in Morlando et al. [16] The FUS–G48A mutant construct was obtained by inverse PCR amplification on FUS– WT plasmid (SC320263, OriGene Technologies) using the oligonucleotides FUS–G48A forward (FW) and reverse (REV), while the FUS-Δ3′-UTR mutant construct was generated by PCR amplification on FUS– WT plasmid using the oligonuclotides FUS-Δ3′-UTR FW and REV. HA–FUS–WT and HA–FUS–G48A were generated by insertion of the HA tag in both FUS– WT and FUS– G48A plasmids through a reverse PCR using the HA-5′FUS FW and REV oligonucleotides. To generate the constructs for the luciferase assay Luc–FUS– WT , the genomic fragment containing the 3′-UTR was PCR amplified using the oligonucleotides FUS-3′-UTR NotI FW and FUS-3′-UTR NotI REV and cloned downstream the Renilla Luciferase open-reading frame in psiCHECK2 vector (Promega) using Not I restriction sites. The mutant derivatives Luc–FUS -Δseed and Luc–FUS– G48A were obtained by inverse PCR amplification using the oligonucleotides FUS 3'-UTR Δseed FW and REV, and FUS–G48A FW and REV, respectively. For the rescue experiment, a 164-nt-long 3′-UTR carrying the G48A substitution was used. This was generated by inverse PCR amplification on Luc–FUS– G48A construct using the FUS–G48A short FW and REV oligonucleotides. Protein extraction and western blot Whole-cell protein extracts were prepared from SK-N-BE cells lysed in RIPA buffer and subjected to western blot analysis performed as previously described [27] . The nuclear/cytoplasmic fractionation was carried out by using the NE-Per Kit (Pierce-Thermo scientific) following the manufacturer’s specifications. The immunoblots were incubated with the following antibodies diluted in 5% skim milk in TBS-T: anti-FUS/TLS (sc-47711, Santa Cruz, 1:2,000), anti-Zeb1 (sc-10572, Santa Cruz, 1:500), anti-HA (sc-7392 Santa Cruz, 1:1,000), anti-Sp1(sc-59 Santa Cruz, 1:1,000) and anti-GAPDH (sc-32233, Santa Cruz, 1:3,000) as a loading control. All the images were captured using the Molecula Imager ChemiDoc XRS + (Bio-Rad), and the densitometric analyses were performed using the associated Image Lab software (Bio-Rad). Luciferase assay Luc–FUS– WT, Luc–FUS -Δseed and Luc–FUS– G48A plasmids were co-transfected with the plasmids expressing miR-141/200a and their mutant derivatives in SK-N-BE cells. After 48 h of incubation, cells were assayed with the Dual-Luciferase Assay (Promega). RNA preparation and analysis Total RNA was isolated using miRNeasy Mini Kit according to the manufacturer’s instructions (Qiagen). 3′-RACE was performed on 2 μg of SK-N-BE total RNA using the FirstChoice RLM-RACE Kit (Ambion) following the manufacturer’s instructions. For miRNA detection, either miScript Reverse Transcription and SYBR-Green PCR Kits [28] or Exiqon miRCURY cDNA synthesis kit together with ExiLENT SYBR Green with Exiqon LNA probes were used. The values obtained were normalized for snoRNA-U25 or snoRNA-U44. For the pri-miRNAs and mRNAs detection the SuperScript VILO cDNA synthesis kit was used. The quantitative reverse transcriptase-PCR was performed with the SYBR-Green PCR Kit (Qiagen) and the oligonucleotides are listed in Supplementary Table 1 . For the detection of the skipping of exon 7, oligonucleotides specific for the isoform lacking the exon 7 (FUS exon 6 FW and FUS exon 6–8 REV) were used. Band-shift Band-shift assays were carried out with minor modifications with respect to the basic protocol [29] . In particular, pri-miRNA substrates were prepared by in vitro transcription, using T7 RNA polymerase (Promega), from PCR-amplified templates (oligonucleotides are listed in Supplementary Table 1 ) in the presence of [α- 32 P]UTP (Perkin-Elmer). The 32 P-labelled RNA transcripts (40,000 c.p.m.) were incubated with 6 nmol of recombinant GST or GST–FUS proteins in the presence of cold transfer RNA competitor for 20 min at room temperature in electrophoretic mobility-shift assay buffer (containing 0.5 μg μl −1 bovine serum albumin, 100 ng μl −1 Escherichia coli transfer RNA, 10 mM Tris pH 7.5, 20 mM EDTA, 1 mM dithiothreitol, 5% glycerol and 2U μl −1 RNasin Plus RNase inhibitor from Promega) in 10 μl reaction. After addition of 4 μl of glycerol 30%, the sample is immediately analysed by a 4% acrylamide non-denaturing gel in tris-borate-EDTA 0.5 × . After drying, the gel is analysed by autoradiograph, and densitometric analysis was performed using the Typhoon Imager (GE Healthcare) and ImageQuant software (Molecular Dynamics). Chromatin immunoprecipitation assay Chromatin immunorecipitation analyses were performed on chromatin extracts from SK-N-BE cells according to manufacturer’s specifications of the MAGnify Chromatin Immunoprecipitation System kit (Invitrogen). Sheared chromatin was immunoprecipitated with anti-FUS/TLS antibody (sc-47711, Santa Cruz). The occupancy of the immunoprecipitated factor on miRNA loci was estimated by normalizing for the occupancy on the chromosome 4 intergenic region and expressed as enrichment over background (immunoglobulin G) [30] . Densitometric analysis was performed using Typhoon Imager (GE Healthcare) and ImageQuant software (Molecular Dynamics). Oligonucleotides used for PCR amplifications are listed in Supplementary Table 1 . Drosha in vitro processing In vitro processing assay was carried out as using labelled pri-miRNA transcripts incubated with 30 μg of SK-N-BE nuclear extract at 37 °C for 90 min in the presence of either 6 nmol of recombinant GST protein or 3 and 6 nmol of recombinant GST–FUS protein [31] . After the incubation, processed RNAs were precipitated and resuspended in 7.5 μl of RNA-loading buffer, heated at 95 ° for 5 min and then separated on a 12.5% urea-polyacrylamide gel. How to cite this article: Modigliani, S. D. et al. An ALS-associated mutation in the FUS 3′-UTR disrupts a microRNA–FUS regulatory circuitry. Nat. Commun. 5:4335 doi: 10.1038/ncomms5335 (2014).